N-acetylglucosamine sensing by a GCN5-relatedN-acetyltransferase induces transcription via chromatin histone acetylation in fungi N-acetylglucosamine (GlcNAc) exists ubiquitously as a component of the surface on a wide range of cells, from bacteria to humans. Many fungi are able to utilize environmental GlcNAc to support growth and induce cellular development, a property important for their survival in various host niches. However, how the GlcNAc signal is sensed and subsequently transduced is largely unknown. Here, we identify a gene that is essential for GlcNAc signalling ( NGS1 ) in Candida albicans , a commensal and pathogenic yeast of humans. Ngs1 can bind GlcNAc through the N-terminal β-N- acetylglucosaminidase homology domain. This binding activates N -acetyltransferase activity in the C-terminal GCN5-related N -acetyltransferase domain, which is required for GlcNAc-induced promoter histone acetylation and transcription. Ngs1 is targeted to the promoters of GlcNAc-inducible genes constitutively by the transcription factor Rep1. Ngs1 is conserved in diverse fungi that have GlcNAc catabolic genes. Thus, fungi use Ngs1 as a GlcNAc-sensor and transducer for GlcNAc-induced transcription. N-acetylglucosamine (GlcNAc) is a major structural component on the cell surface of a wide range of cells [1] . It is a component of the peptidoglycan of bacterial cell walls and the extracellular matrix glycosaminoglycans of animal cells. The polymer of GlcNAc, chitin, is a component of fungal cell walls and exoskeletons of arthropods such as crustaceans and insects. The GlcNAc released from these polymers is taken up and used by microbes. In bacteria, GlcNAc regulates the expression of GlcNAc synthesis and catabolic genes, virulence properties [1] , as well as cellular development and antibiotic production [2] . In fungi, GlcNAc induces GlcNAc catabolic genes and morphogenesis programs. Uptake and intracellular catabolism of GlcNAc have been mostly studied in Candida albicans , the major pathogenic yeast of humans. GlcNAc enters C. albicans cells by a plasma membrane transporter, Ngt1 (ref. 3 ). Intracellular GlcNAc induces the expression of three GlcNAc catabolic genes: GlcNAc kinase (Hxk1), GlcNAc-6-phosphate deacetylase (Dac1), and GlcN-6-phosphate deaminase (Nag1), all of which act sequentially to convert GlcNAc to fructose-6-phosphate which is then fed into the glycolytic pathway. The catabolic genes and NGT1 are conserved in fungi [4] , [5] , [6] . Recently, a transcription factor was found to control the expression of GlcNAc catabolic genes in the filamentous fungus Trichoderma reesei [6] . Although some metabolites have been shown to activate gene expression through direct modulation of transcription factors in unicellular organisms [7] , little is known about the mechanism of how GlcNAc is sensed and how the signal is transduced to induce the expression of its catabolic genes in fungi. The lack of GlcNAc catabolic genes in Saccharomyces cerevisiae and Schizosaccharomyces pombe has hindered the discovery of a GlcNAc signalling pathway in fungi. Chemical modifications of histones, such as methylation and acetylation, play critical roles in epigenetic gene regulation. Many of the enzymes that add or remove such chemical modifications are known to be sensitive to changes in intracellular metabolism. By neutralizing the positive charge of histone tails, acetylation serves to loosen histone-DNA interactions and allow transcription factors to access promoter chromatin [8] . Chromatin acetylation also provides binding sites for effector proteins to recruit coactivators for transcription [9] . Histone acetylation is established by the opposing functions of histone acetyltransferase (HAT) and deacetylase (HDAC) enzymes. Gcn5 was the first HAT that was discovered and extensively studied [10] . Structural studies of members of the superfamily of GCN5-related N -acetyltransferases (GNATs) provided the first atomic resolution structures of HATs for conserved mechanisms of acetyl-CoA interaction [11] . Enzymatic activities of HATs are regulated by phosphorylation, interaction with other proteins [10] , and the metabolic state of the cell [12] . However, the link between metabolic substrates and their ability to directly influence epigenetic signalling remains incompletely understood. As a part of the commensal microbiota, C. albicans colonizes multiple mucosal sites, including the gastrointestinal (GI) tract. GlcNAc has been implicated in commensal growth of C. albicans in the GI tract [13] , where glucose is often limited and GlcNAc can be released from bacteria. C. albicans can also scavenge GlcNAc from glycosaminoglycan of the host cell extracellular matrix by secreting a GlcNAc-inducible β-hexosaminidase [14] . The ability to use environmental GlcNAc is important for the existence of C. albicans in its host niches, as GlcNAc catabolic pathway mutants have significantly reduced virulence [15] , [16] , [17] . Not only can GlcNAc induce genes for GlcNAc catabolism, it can also promote C. albicans cells to undergo hyphal development [18] and phenotypic switching between two heritable cell states [19] . These morphogenesis programs of C. albicans are linked to its virulence, infection of distinct host niches and immune evasion [20] , [21] . In addition to C. albicans , GlcNAc also triggers a rapid morphogenetic programme in two thermally dimorphic fungal pathogens, Histoplasma capsulatum and Blastomyces dermatitidis [4] . Uncovering the mechanism for GlcNAc signalling is important for understanding fungal pathogenesis. Here we report a gene that is required for N-acetylglucosamine signalling ( NGS1 ) and catabolism. Ngs1 contains a conserved GlcNAc binding pocket at its N-terminus and a C-terminal GNAT domain; both are important for GlcNAc-induced promoter chromatin acetylation and transcription of GlcNAc catabolic genes. Ngs1 also controls other GlcNAc-induced transcription programs and is conserved in diverse fungi. Thus, Ngs1 is a novel GlcNAc signal sensor-transducer in fungi. Identifying a novel protein essential for GlcNAc signalling To uncover the GlcNAc signalling pathway, we performed a genetic screen with C. albicans deletion libraries for mutants defective in growth on GlcNAc as the sole carbon source. None of the 165 transcriptional factors [22] and none of the 80 kinases and kinase-related genes [23] is required for growth on GlcNAc. From a knockout library of 674 unique genes in C. albicans [24] , three mutants ( nag1, snf4, orf19.7516 ( CR_00190W )) were found to be unable to grow on GlcNAc ( Fig. 1a ). orf19.7516 is specifically required for GlcNAc utilization as the orf19.7516 mutant grew well on galactose or on GlcNAc media supplemented with galactose or amino acids, similar to the GlcNAc transporter mutant ngt1 (ref. 3 ). Snf4 is not specific for GlcNAc signalling as it is also required for growth on galactose, consistent with its function in S. cerevisiae for metabolizing alternative carbon sources in the absence of glucose [25] . As reported, the nag1 showed a growth defect on all GlcNAc containing media, even when supplemented with galactose or amino acids, due to GlcNAc-6-PO 4 accumulation that is suggested to inhibit the growth of C. albicans cells [26] . We also screened the GRACE library, a non-redundant library containing a total of 2,357 different mutants [27] . ngt1 and orf19.7516 were the only two mutants found specifically defective in GlcNAc utilization from the GRACE library and the deletion libraries we screened, which cover about 40% genes in the genome. 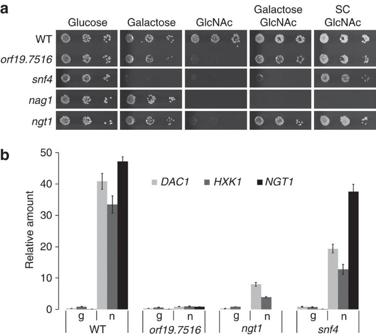Figure 1:ngs1(orf19.7516) andngt1are specifically defective in GlcNAc signalling and catabolism. (a) Cells of wild-type (SN250),orf19.7516, snf4, nag1andngt1(HLY4394) mutant strains were serially diluted 10-fold and spotted onto YNB solid medium containing 2.5 mM of the indicated sugar or SC solid medium containing 2.5 mM GlcNAc. The YNB medium was supplemented with 0.1 mg ml−1arginine to permit growth. Photographs were taken after 2 days of growth at 30 °C. (b) qRT-PCR analysis of GlcNAc catabolic genesDAC1andHXK1and GlcNAc transporterNGT1upon GlcNAc induction in the wild type (SN250) and indicated mutants. Cells were grown in liquid SC medium with 2.5 mM GlcNAc (n) or 5% glycerol (g) for 2 h at 30 °C for RNA extraction. Mean data±s.d. from three independent qRT-PCR experiments was plotted. Figure 1: ngs1 ( orf19.7516 ) and ngt1 are specifically defective in GlcNAc signalling and catabolism. ( a ) Cells of wild-type (SN250), orf19.7516, snf4, nag1 and ngt1 (HLY4394) mutant strains were serially diluted 10-fold and spotted onto YNB solid medium containing 2.5 mM of the indicated sugar or SC solid medium containing 2.5 mM GlcNAc. The YNB medium was supplemented with 0.1 mg ml −1 arginine to permit growth. Photographs were taken after 2 days of growth at 30 °C. ( b ) qRT-PCR analysis of GlcNAc catabolic genes DAC1 and HXK1 and GlcNAc transporter NGT1 upon GlcNAc induction in the wild type (SN250) and indicated mutants. Cells were grown in liquid SC medium with 2.5 mM GlcNAc (n) or 5% glycerol (g) for 2 h at 30 °C for RNA extraction. Mean data±s.d. from three independent qRT-PCR experiments was plotted. Full size image To determine if the orf19.7516 mutant is defective in GlcNAc signalling, we examined whether GlcNAc catabolic genes or the transporter NGT1 are induced. ORF19.7516 was essential for the induction of HXK1, DAC1 and NGT1 in response to GlcNAc ( Fig. 1b ). Therefore, we designate ORF19.7516 as NGS1 for N-acetylglucosamine signalling. Intracellular GlcNAc is responsible for GlcNAc signalling in C albicans [26] ; however, we detected a slight increase in HXK1 and DAC1 expression in the ngt1 mutant, which could be attributed to the existence of a low affinity GlcNAc uptake process [3] , [28] . The essential function of Ngs1 in GlcNAc signalling is not due to its requirement for NGT1 expression and GlcNAc transport because ectopic expression of NGT1 could not bypass the growth defect of the ngs1 mutant on GlcNAc ( Supplementary Fig. 1a ). The growth defect of the ngs1 mutant on GlcNAc could be rescued by reintroducing a copy of NGS1 under its own promoter or an N-terminally FLAG-tagged Ngs1 ( Supplementary Fig. 1a ). Ngs1 levels were similar in cells grown in glucose or GlcNAc ( Supplementary Fig. 2a,b ), suggesting that GlcNAc signalling is not mediated by changing Ngs1 levels. GlcNAc binding with Ngs1 is essential for GlcNAc signalling NGS1 encodes an uncharacterized protein of 963 amino acids. The N-terminus of Ngs1 contains high conservation to β-N- acetylglucosaminidases in the Glycoside Hydrolase family 3 (GH3) [29] , which exhibit unique substrate specificity for GlcNAc [30] ( Fig. 2a,b ). The C-terminal region of Ngs1 has a weak homology to the N -Acyltransferase (NAT) domain in the GCN5-related N -acetyltransferase (GNAT) family [31] , [32] ( Fig. 2a ). In front of the NAT domain lays a putative nuclear localization signal (NLS), predicted by cNLS Mapper [33] ( Fig. 2a ). The two putative, functionally distinct domains of Ngs1 are both required for Ngs1 function, as expressing the N-terminus (aa 1–341) or C terminus (aa 341–963) of Ngs1 was insufficient to complement the growth defect of ngs1 on GlcNAc ( Supplementary Figs 1a and 3a ). 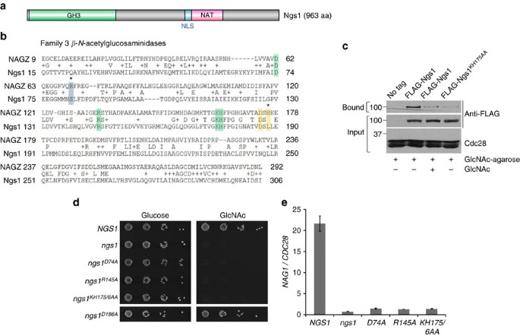Figure 2: Binding of GlcNAc to Ngs1 is required for GlcNAc signalling. (a) Schematic depiction of the Glycoside Hydrolase family 3 (GH3) domain (green box),N-Acyltransferase (NAT) domain (pink box), and nuclear localization signal (NLS) region (blue box) in Ngs1. (b) Sequence alignment of the GH3β-N-acetylglucosaminidase domain between Ngs1 andStNagZ. The residues known to interact with GlcNAc (boxed in green) or anhMurNAc (boxed in blue), and the Asp-His dyad involved in catalysis (boxed in yellow) are indicated. Residues divergent in Ngs1 are indicated by asterisks. (c) Binding of Ngs1 to GlcNAc-agarose beads. Protein extracts from thengs1mutants expressing untagged Ngs1 (HLY4395), FLAG-tagged Ngs1 (HLY4402), or FLAG-tagged Ngs1KH175/6AA(HLY4405) were incubated with GlcNAc-agarose at 4 °C overnight in the absence or presence of 100 mM GlcNAc. The input and bound fractions were analysed on Western blots probed with FLAG antibody. (d) Mutations in the GlcNAc binding sites of Ngs1 abolished growth on GlcNAc.ngs1mutant cells carrying a wild-type copy ofNGS1(HLY4395),ngs1D74A(HLY4398),ngs1R145A(HLY4399),ngs1KH175/6AA(HLY4400),ngs1D186A(HLY4401) or vector alone (HLY4396) were serially diluted 10-fold and spotted onto YNB solid medium containing 2.5 mM GlcNAc or glucose. Colony growth was assessed after 2 days of growth at 30 °C. (e) GlcNAc could not induceNAG1expression in strains carrying mutations in GlcNAc binding sites in Ngs1. Cells were grown in liquid SC medium with 2.5 mM GlcNAc for 2 h at 30 °C for RNA extraction. All data showed the average of three independent qRT-PCR experiments with error bars representing the s.d. Figure 2: Binding of GlcNAc to Ngs1 is required for GlcNAc signalling. ( a ) Schematic depiction of the Glycoside Hydrolase family 3 (GH3) domain (green box), N- Acyltransferase (NAT) domain (pink box), and nuclear localization signal (NLS) region (blue box) in Ngs1. ( b ) Sequence alignment of the GH3 β-N- acetylglucosaminidase domain between Ngs1 and St NagZ. The residues known to interact with GlcNAc (boxed in green) or anhMurNAc (boxed in blue), and the Asp-His dyad involved in catalysis (boxed in yellow) are indicated. Residues divergent in Ngs1 are indicated by asterisks. ( c ) Binding of Ngs1 to GlcNAc-agarose beads. Protein extracts from the ngs1 mutants expressing untagged Ngs1 (HLY4395), FLAG-tagged Ngs1 (HLY4402), or FLAG-tagged Ngs1 KH175/6AA (HLY4405) were incubated with GlcNAc-agarose at 4 °C overnight in the absence or presence of 100 mM GlcNAc. The input and bound fractions were analysed on Western blots probed with FLAG antibody. ( d ) Mutations in the GlcNAc binding sites of Ngs1 abolished growth on GlcNAc. ngs1 mutant cells carrying a wild-type copy of NGS1 (HLY4395), ngs1 D74A (HLY4398), ngs1 R145A (HLY4399), ngs1 KH175/6AA (HLY4400), ngs1 D186A (HLY4401) or vector alone (HLY4396) were serially diluted 10-fold and spotted onto YNB solid medium containing 2.5 mM GlcNAc or glucose. Colony growth was assessed after 2 days of growth at 30 °C. ( e ) GlcNAc could not induce NAG1 expression in strains carrying mutations in GlcNAc binding sites in Ngs1. Cells were grown in liquid SC medium with 2.5 mM GlcNAc for 2 h at 30 °C for RNA extraction. All data showed the average of three independent qRT-PCR experiments with error bars representing the s.d. Full size image A pivotal question is whether the intracellular GlcNAc signal is transmitted via the GH3 β-N- acetylglucosaminidase homology domain. The N-terminal region of Ngs1 (aa 15–306) is most similar to bacterial NagZs with 28% identity to Salmonella typhimurium NagZ ( Fig. 2b ). The GH3 NagZ enzymes participate in bacterial cell wall recycling by removing terminal GlcNAc from GlcNAc-anhMurNAc-peptide in Gram-negative bacteria [34] and GlcNAc-MurNAc-peptide in Gram-positive bacteria [35] . Crystal structure determinations of NagZ enzymes in complex with their natural substrates (for example, GlcNAc-anhMurNAc) and its product GlcNAc have defined binding coordinates/residues of the NagZ family of enzymes for GlcNAc and anhMurNAc [36] . The conserved key GlcNAc binding sites in St NagZ are also present in Ngs1 ( Fig. 2b , green shade), whereas the binding site for the lactyl moiety of anhMurNAc is divergent in Ngs1 ( Fig. 2b , blue shade) [36] , which suggest that Ngs1 has GlcNAc monomer binding sites, but has lost the binding pocket for the disaccharide GlcNAc-anhMurNAc. In support of the sequence conservation, agarose conjugated with GlcNAc was able to pull down FLAG-Ngs1 ( Fig. 2c ). The binding of GlcNAc-agarose with FLAG-Ngs1 was greatly reduced when free GlcNAc was added to the cell lysate before incubation with GlcNAc-agarose. The interaction was also disrupted by mutating the conserved GlcNAc binding residues K175H176 in the GH3 domain of Ngs1. Thus, Ngs1 can bind GlcNAc via the conserved GlcNAc binding pocket. We further showed that the GlcNAc binding sites in Ngs1 are critical for its function in GlcNAc signalling, as mutations in the conserved residues D74, R145 and K175H176 resulted in a dramatic growth defect on GlcNAc ( Fig. 2d ). Addition of GlcNAc could not induce the expression of catabolic genes in these mutants ( Fig. 2e ). Mutating the GlcNAc binding sites did not affect their expression ( Supplementary Fig. 3b ). Altogether, our data suggested that Ngs1 can bind GlcNAc, and this binding is important for its function of sensing intracellular GlcNAc. Ngs1 is able to sense GlcNAc at micromolar levels and induce GlcNAc catabolic genes within minutes ( Supplementary Fig. 4 ). Since Ngs1 is highly homologous to GH3 β-N- acetylglucosaminidase, one obvious question is whether Ngs1 is a hydrolase. Most NagZ enzymes from Gram-negative bacteria are single domain enzymes and their catalytic domain contains the conserved aspartate nucleophile and a catalytic histidine/aspartate dyad [29] , [36] ( Fig. 2b , shaded in yellow). The conserved Asp-His dyad of NagZs are essential for the catalytic reaction of this family of enzymes. However, the histidine in the Asp-His dyad of NagZ is replaced by a leucine in Ngs1. Also, replacement of the Asp186 with alanine did not affect Ngs1′s function ( Fig. 2d ). Therefore, we suggest that Ngs1 is not a hydrolase. Consistent with this notion, we could not detect N -acetylglucosaminidase activity in an affinity pull-down of FLAG-Ngs1 from C. albicans cells grown in GlcNAc. Thus, the GlcNAc binding ability, but not hydrolase activity, is important for Ngs1's function in GlcNAc signalling. Ngs1 is associated with promoters of GlcNAc catabolic genes The rapid response to GlcNAc indicates that regulators in the GlcNAc signalling pathway are preexisting. Indeed, Ngs1 protein levels are unchanged before or after GlcNAc induction ( Supplementary Fig. 2a ). Functional GFP-Ngs1 expressed from the MAL2 promoter ( Supplementary Fig. 5 ) accumulated in the nucleus in the absence or presence of GlcNAc ( Fig. 3a ). To determine if Ngs1 is present at the promoters of its target genes, functional N-terminal FLAG-tagged Ngs1 was used to determine its association at the divergent promoter region shared by NAG1 and DAC1 by chromatin immunoprecipitation. Ngs1 was found associated with the promoter in a GlcNAc-independent manner ( Fig. 3b ). Therefore, Ngs1 functions at the promoter of GlcNAc catabolic genes to activate transcription in response to GlcNAc. 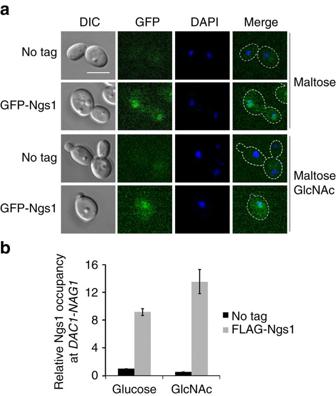Figure 3: Ngs1 binds to the promoter of GlcNAc catabolic genes. (a) Thengs1mutant strain expressing GFP-Ngs1 under theMAL2promoter (HLY4397) was grown to log phase in liquid SC medium containing 50 mM maltose at 30 °C, and then treated with or without 50 mM GlcNAc for 30 min. Cell morphology and Ngs1 localization were observed by using DIC and fluorescence microscopy. An untagged control (SC5314) was included. For all images: Scale bar, 5 μm. (b) Ngs1 is present at the promoter forNAG1andDAC1in a GlcNAc-independent manner. Overnight cultures ofngs1mutant cells carrying 3FLAG-Ngs1 (HLY4402) or untagged Ngs1 (HLY4395) from theNGS1promoter were pelleted, washed three times in PBS, diluted 1:20 in SC medium with 10 mM GlcNAc or glucose at 30 °C, and cells were collected at 30 min for the ChIP experiment. ChIP DNA was quantitated as described64by qPCR with primers at the promoter region ofNAG1andDAC1. TheACT1promoter region was used as a control. The enrichment is presented as a ratio ofNAG1-DAC1promoter IP (bound/input) versusACT1promoter IP (bound/input). The value inngs1mutant cells carrying untagged Ngs1 (HLY4395) in glucose medium was set to 1.00. The ChIP data showed the average of three independent qPCR data with error bars representing the s.d. Figure 3: Ngs1 binds to the promoter of GlcNAc catabolic genes. ( a ) The ngs1 mutant strain expressing GFP-Ngs1 under the MAL2 promoter (HLY4397) was grown to log phase in liquid SC medium containing 50 mM maltose at 30 °C, and then treated with or without 50 mM GlcNAc for 30 min. Cell morphology and Ngs1 localization were observed by using DIC and fluorescence microscopy. An untagged control (SC5314) was included. For all images: Scale bar, 5 μm. ( b ) Ngs1 is present at the promoter for NAG1 and DAC1 in a GlcNAc-independent manner. Overnight cultures of ngs1 mutant cells carrying 3FLAG-Ngs1 (HLY4402) or untagged Ngs1 (HLY4395) from the NGS1 promoter were pelleted, washed three times in PBS, diluted 1:20 in SC medium with 10 mM GlcNAc or glucose at 30 °C, and cells were collected at 30 min for the ChIP experiment. ChIP DNA was quantitated as described [64] by qPCR with primers at the promoter region of NAG1 and DAC1 . The ACT1 promoter region was used as a control. The enrichment is presented as a ratio of NAG1-DAC1 promoter IP (bound/input) versus ACT1 promoter IP (bound/input). The value in ngs1 mutant cells carrying untagged Ngs1 (HLY4395) in glucose medium was set to 1.00. The ChIP data showed the average of three independent qPCR data with error bars representing the s.d. Full size image The HAT activity in Ngs1 GNAT domain The C-terminal region of Ngs1 is essential for growth on GlcNAc and contains a weak sequence homology to the NAT domain of the GCN5-related N -acetyltransferase (GNAT) family [31] , [32] . GNAT members are known to share weak similarities by sequence alignment, but they all have a universally conserved secondary structure [37] , containing a fold comprised of an N-terminal strand followed by two helixes, three β strands, followed by a signature central helix, a fifth β strand, a fourth α helix and a final β strand. The secondary structure is also found in the C-terminal region of Ngs1 using Jpred [38] and PredictProtein [39] ( Fig. 4a ). Members of the GNAT superfamily usually have four conserved motifs A to D [40] . Motif A is the core of the GNAT domain and is conserved in all members. Motif C is missing in some GNATs [9] . Ngs1 contains motifs A, B and D ( Fig. 4a ). The highly conserved residues in motif A are also conserved in Ngs1 ( Fig. 4a ) [32] . The conserved catalytic residue can be either glutamate or histidine ( Fig. 4a , shaded in yellow) [31] , [41] . 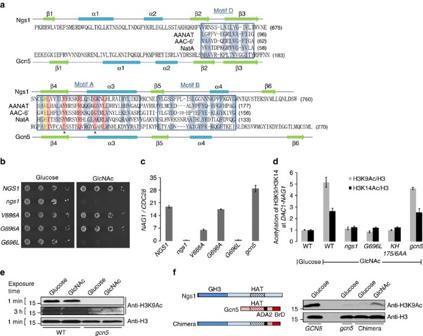Figure 4: Conserved acetyl-CoA interacting residues of Ngs1 are required for GlcNAc-induced promoter histone acetylation and transcription. (a) Sequence alignment of GNAT homology motifs A, B, and D in Ngs1 andC. albicansGcn5 and three GNAT superfamily members (sheep AANAT, arylalkylamine-N-acetyltransferase68;Enterococcus faeciumAAC-6′, aminoglycoside 6′-N-acetyltransferase32;S. pombeNatA,N-acetyltransferase complex catalytic subunit57). Consensus residues throughout the superfamily, as determined by Neuwald and Landsman40, are shown with blue shade, and residues particularly conserved in motif A are shaded in pink. The yellow shade indicates the residue known to be critical for HAT catalysis inTetrahymenaGcn5. The asterisks under the aligned sequences show the location of residues known to interact with the Acetyl-CoA. Secondary structure elements of Ngs1 and Gcn5 fromC. albicansare also shown. (b) Dilutions ofngs1mutant cells carryingNGS1(HLY4395),ngs1V686A(HLY4406),ngs1G696A(HLY4407),ngs1G696L(HLY4408), or vector alone (HLY4396) were spotted onto the solid YNB media plates containing 2.5 mM GlcNAc or glucose and then incubated at 30 °C for 2 days. (c)NAG1mRNA levels of the strains from (b) and thegcn5mutant (CPS50) were determined in GlcNAc-containing medium by qRT-PCR. (d) ChIP with anti-H3, anti-acetylated H3K9, and anti-acetylated H3K14 antibodies in the wild type (SN250),ngs1mutant cells carryingngs1G696L(HLY4408),ngs1KH175/6AA(HLY4400) or vector alone (HLY4396), andgcn5mutant cells carrying vector (CPS50). Cells were grown in GlcNAc or glucose for 30 min for the ChIP experiment. The value from wild type in glucose medium was set to 1.00. (e) Global H3K9 acetylation level is not induced by GlcNAc. Cell lysates of wild type (SN250) andgcn5mutant (CPS50) growing in GlcNAc or glucose medium were subjected to Western analysis. (f) GlcNAc regulated H3K9 acetylation by the Ngs1-Gcn5 chimera in thegcn5mutant. Thegcn5revertant andgcn5mutant carrying the empty vector or chimeric construct were grown overnight in YEP containing 100 mM GlcNAc or glucose at 30 °C to saturation for Western analysis. The construct is schematically illustrated on the left (ADA2, ADA2 interaction domain; BrD, bromodomain). Mean data±s.d. from three independent qPCR experiments was plotted. Figure 4: Conserved acetyl-CoA interacting residues of Ngs1 are required for GlcNAc-induced promoter histone acetylation and transcription. ( a ) Sequence alignment of GNAT homology motifs A, B, and D in Ngs1 and C. albicans Gcn5 and three GNAT superfamily members (sheep AANAT, arylalkylamine- N -acetyltransferase [68] ; Enterococcus faecium AAC-6′, aminoglycoside 6′- N -acetyltransferase [32] ; S. pombe NatA, N -acetyltransferase complex catalytic subunit [57] ). Consensus residues throughout the superfamily, as determined by Neuwald and Landsman [40] , are shown with blue shade, and residues particularly conserved in motif A are shaded in pink. The yellow shade indicates the residue known to be critical for HAT catalysis in Tetrahymena Gcn5. The asterisks under the aligned sequences show the location of residues known to interact with the Acetyl-CoA. Secondary structure elements of Ngs1 and Gcn5 from C. albicans are also shown. ( b ) Dilutions of ngs1 mutant cells carrying NGS1 (HLY4395), ngs1 V686A (HLY4406), ngs1 G696A (HLY4407), ngs1 G696L (HLY4408), or vector alone (HLY4396) were spotted onto the solid YNB media plates containing 2.5 mM GlcNAc or glucose and then incubated at 30 °C for 2 days. ( c ) NAG1 mRNA levels of the strains from ( b ) and the gcn5 mutant (CPS50) were determined in GlcNAc-containing medium by qRT-PCR. ( d ) ChIP with anti-H3, anti-acetylated H3K9, and anti-acetylated H3K14 antibodies in the wild type (SN250), ngs1 mutant cells carrying ngs1 G696L (HLY4408), ngs1 KH175/6AA (HLY4400) or vector alone (HLY4396), and gcn5 mutant cells carrying vector (CPS50). Cells were grown in GlcNAc or glucose for 30 min for the ChIP experiment. The value from wild type in glucose medium was set to 1.00. ( e ) Global H3K9 acetylation level is not induced by GlcNAc. Cell lysates of wild type (SN250) and gcn5 mutant (CPS50) growing in GlcNAc or glucose medium were subjected to Western analysis. ( f ) GlcNAc regulated H3K9 acetylation by the Ngs1-Gcn5 chimera in the gcn5 mutant. The gcn5 revertant and gcn5 mutant carrying the empty vector or chimeric construct were grown overnight in YEP containing 100 mM GlcNAc or glucose at 30 °C to saturation for Western analysis. The construct is schematically illustrated on the left (ADA2, ADA2 interaction domain; BrD, bromodomain). Mean data±s.d. from three independent qPCR experiments was plotted. Full size image To determine if the predicted N -acetyltransferase activity in Ngs1 is required for GlcNAc signalling, point mutations were introduced to the residues that are known to interact with Acetyl-CoA in GNATs ( Fig. 4a , asterisk mark) [32] . Val686 and Gly696 were substituted with alanine. We also mutated Gly696 to leucine because several GNATs have alanine instead of glycine at this position [42] . The function of each mutant Ngs1 was tested in the ngs1 mutant. The ngs1 G696L mutant could not grow on GlcNAc like the ngs1 deletion mutant ( Fig. 4b ), and was unable to express NAG1 in response to GlcNAc ( Fig. 4c ). In addition, cells carrying the V686A mutation showed impaired induction of NAG1 . The protein levels of both ngs1 G696L and ngs1 V686A are largely unchanged compared to that of wild-type Ngs1 ( Supplementary Fig. 3c ). The G696A mutaion had no detectable phenotype as expected. Thus, the conserved acetyl-CoA interacting residues in the predicted N -acetyltransferase domain of Ngs1 are essential for GlcNAc signalling. GNATs catalyse the transfer of an acetyl group from Acetyl-CoA to the amine of a wide range of substrates, including small molecules and proteins. For example, AANAT, NatA and AAC-6′ acetylate arylakylamine, protein N-terminal or aminoglucoside, respectively. The founding member Gcn5 functions as a coactivator that facilitates initiation of transcription by acetylating N-terminal lysines on H3 (ref. 10 ). We reasoned that this could be a possible mechanism for how promoter-associated Ngs1 regulates transcription upon GlcNAc induction. By immunoprecipitation with anti-acetylated-H3K9 antibodies, we observed a dramatic increase in the level of acetylated H3K9 at the promoter region of DAC1 and NAG1 in wild-type cells within 30 min of GlcNAc induction ( Fig. 4d ), in agreement with the role of H3K9ac in transcriptional initiation [43] , [44] . An increase in the level of H3K14ac was also observed upon addition of GlcNAc, albeit the fold of increase was lower than that of H3K9ac. Importantly, the GlcNAc-induced increase in H3K9 and H3K14 acetylation was abolished in the ngs1 deletion mutant or ngs1 G696L mutant ( Fig. 4d ), suggesting an essential role of the N -acetyltransferase domain of Ngs1 for its function in histone acetylation in response to GlcNAc. The C. albicans Gcn5, a homologue of S. cerevisiae Gcn5, is a major HAT for histone H3 acetylation in C. albicans [45] . Consistent with this notion, we found that acetylation at H3K9 is much lower in the gcn5 mutant ( Fig. 4e ). Despite the major role Gcn5 plays in H3K9ac, it is not required for GlcNAc-induced chromatin acetylation of H3K9 and H3K14 or transcription ( Fig. 4c,d ). Therefore, the GlcNAc-induced increase in chromatin H3 acetylation is mediated through the C-terminal GNAT domain of Ngs1 but not Gcn5. However, we cannot detect any increase in the total level of H3K9ac upon GlcNAc induction even in gcn5 mutant cells where the basal level of H3K9ac is low ( Fig. 4e ). ScGcn5 cannot acetylate nucleosomal histones by itself [10] ; its substrate preference is expanded in the context of HAT complexes (Ada and SAGA). Thus the difference of substrate specificity between Gcn5 and Ngs1 is, at least in part, modulated by other proteins within the HAT complexes. ScGcn5 contains a roughly 160-residue HAT domain and an adjacent C-terminal domain that contains an ADA2-interaction domain and a conserved bromodomain, which may provide contact sites for other proteins within the HAT complexes. In order to determine if the GNAT domain in Ngs1 has the predicted HAT activity in response to GlcNAc, the GNAT domain of Gcn5 was replaced by the N-terminus of Ngs1 (1-752 aa, including the GH3 domain and GNAT domain). The chimera failed to increase the acetylation level of H3K9 in gcn5 mutant in glucose, but led to a significant increase in H3K9 acetylation in response to GlcNAc; although it is insufficient to restore the full HAT activity of Gcn5 ( Fig. 4f ). We further showed that mutating the predicted GlcNAc binding sites (K175H176) in Ngs1 blocked GlcNAc-induced acetylation on promoter chromatin H3K9 and H3K14 ( Fig. 4d ). Therefore, our data demonstrated that GlcNAc binding to the GH3 homology domain of Ngs1 is necessary for its HAT activity of GNAT domain, which is required for GlcNAc signalling. Conservation of Ngs1 in diverse fungi We performed BLAST searches to analyse the distribution of Ngs1 orthologs in fungi and found that Ngs1 orthologs are in many species belonging to the two subphyla, Saccharomycotina and Pezizomycotina , as recently reported [6] . Similar to the conservation of GlcNAc catabolic genes in the Saccharomycotina class, Ngs1 orthologs are found in organisms most closely related to C. albicans and missing in yeast that are more related to S. cerevisiae [3] , [46] . All the Ngs1 orthologs in the Saccharomycotina class carry an N-terminal domain with a high homology to the GH3 β - N -acetylglucosaminidase and a C-terminal region with a weak homology to the NAT domain in the GNAT family ( Fig. 5a ). Like C. albicans Ngs1, the conserved GlcNAc binding residues in the β - N -acetylglucosaminidase domain are present, whereas the Asp-His dyad residues required for the catalytic function and the binding site for the lactyl moiety of anhMurNAc are divergent in the Ngs1 orthologs. BLASTP analysis also identified Ngs1 orthologs throughout many different species of Pezizomycotina, such as Git7 in Histoplasma capsulatum [4] and Nag3 in T. reesei [6] . Interestingly, Ngs1 orthologs are often present in the GlcNAc utilization gene cluster in filamentous fungi (Pezizomycotina) [6] , but Ngs1 is not associated with this cluster in C. albicans . Further, the transcriptional induction by GlcNAc was found for H. capsulatum GIT7 and T. reesei NAG3, but not for C. albicans NGS1 ( Supplementary Fig. 2b ). Ngs1 orthologs in Pezizomycotina contain the highly conserved GH3 domain at the N-terminus and NAT domain at the C-terminus. The GH3 domain carries conserved GlcNAc binding residues ( Fig. 5a , shaded in green) and a glutamate acting as the acid/base catalyst in β –glucosidases subfamily ( Fig. 5a , shaded in yellow) [47] , and therefore may retain the hydrolase activity. The Ngs1 orthologs in Pezizomycotina class are expected to have the ability to recognize GlcNAc monomer and transduce the GlcNAc signal, as deletion of NAG3 in T. reesei resulted in a growth defect on GlcNAc (ref. 6 ). 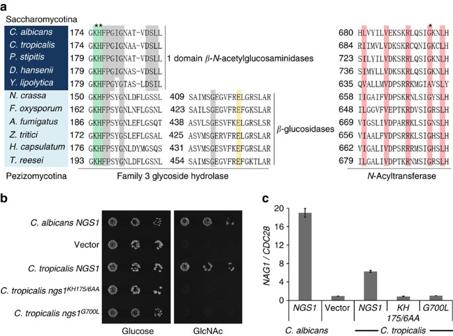Figure 5: Evolutionary conservation of GlcNAc signalling in Ascomycota. (a) Partial multiple sequence alignment of Ngs1 orthologs in the GH3 glycosidase domain and theN-Acyltransferase domain from Saccharomycotina (shaded in dark blue) and Pezizomycotina (shaded in light blue). The conserved residues in one domainβ-N-acetylglucosaminidases and two domainβ-glucosidases, as determined by Litzinger and Fischer29, are shaded in grey. The residues known to interact with GlcNAc (shaded in green) and the glutamate residue known to act as the acid/base catalyst inβ–glucosidases subfamily (shaded in yellow) are indicated. Residues shaded in pink in theN-Acyltransferase domain are conserved in motif A, as shown inFig. 4a. The asterisks indicate the positions used in the mutational analysis inC. tropicalis.(b) Ectopically expressedCtNGS1suppresses the growth defect ofCangs1mutant on GlcNAc. Dilutions ofC. albicans ngs1mutant cells carryingCaNGS1(HLY4395),CtNGS1(HLY4456),Ctngs1KH175/6AA(HLY4457),Ctngs1G700L(HLY4458) or vector alone were grown on YNB plates containing 2.5 mM GlcNAc or glucose at 30 °C for 2 days. (c) The conserved key GlcNAc binding sites K175H176 and acetyl-CoA interacting residue G700 in CtNgs1 are required for the induction ofNAG1inC. albicans.NAG1mRNA levels of the strains from (b) were determined. Cells were grown in liquid SC medium supplemented with 2.5 mM GlcNAc at 30 °C and collected at 15 min for qRT-PCR analysis. Mean data±s.d. from three independent qRT-PCR experiments was plotted. Figure 5: Evolutionary conservation of GlcNAc signalling in Ascomycota. ( a ) Partial multiple sequence alignment of Ngs1 orthologs in the GH3 glycosidase domain and the N- Acyltransferase domain from Saccharomycotina (shaded in dark blue) and Pezizomycotina (shaded in light blue). The conserved residues in one domain β-N- acetylglucosaminidases and two domain β -glucosidases, as determined by Litzinger and Fischer [29] , are shaded in grey. The residues known to interact with GlcNAc (shaded in green) and the glutamate residue known to act as the acid/base catalyst in β –glucosidases subfamily (shaded in yellow) are indicated. Residues shaded in pink in the N- Acyltransferase domain are conserved in motif A, as shown in Fig. 4a . The asterisks indicate the positions used in the mutational analysis in C. tropicalis. ( b ) Ectopically expressed CtNGS1 suppresses the growth defect of Cangs1 mutant on GlcNAc. Dilutions of C. albicans ngs1 mutant cells carrying CaNGS1 (HLY4395), CtNGS1 (HLY4456), Ctngs1 KH175/6AA (HLY4457), Ctngs1 G700L (HLY4458) or vector alone were grown on YNB plates containing 2.5 mM GlcNAc or glucose at 30 °C for 2 days. ( c ) The conserved key GlcNAc binding sites K175H176 and acetyl-CoA interacting residue G700 in CtNgs1 are required for the induction of NAG1 in C. albicans . NAG1 mRNA levels of the strains from ( b ) were determined. Cells were grown in liquid SC medium supplemented with 2.5 mM GlcNAc at 30 °C and collected at 15 min for qRT-PCR analysis. Mean data±s.d. from three independent qRT-PCR experiments was plotted. Full size image To further determine if the function of Ngs1 orthologs is conserved in fungi, we examined the ability of Candida tropicalis Ngs1 to complement the GlcNAc utilization defect in C. albicans ngs1 mutant. The cross-species experiment showed that ectopically expressed CtNGS1 rescued the growth defect in the Cangs1 mutant on GlcNAc ( Fig. 5b ), and partially rescued the defects in the induction of a GlcNAc catabolic gene ( Fig. 5c ). Furthermore, the conserved GlcNAc binding sites (K175H176) and acetyl-CoA interacting residue (G700) in CtNgs1 are necessary for its function in GlcNAc signalling ( Fig. 5b,c ). Altogether, the results suggest that the Ngs1-mediated GlcNAc sensing and signal transduction is conserved in fungi. Rep1 recruits Ngs1 to promoters The GlcNAc utilization gene cluster in filamentous fungi ( Pezizomycotina ) frequently harbours a transcription factor with an Ndt80-like DNA-binding domain, which is required for GlcNAc-induced expression of catabolic genes in T. reesei , designated as Ron1 (ref. 6 ). Its ortholog in C. albicans is Rep1, a negative regulator of MDR1 transcription [48] . We found that, similar to Ron1 in T. reesei, Rep1 was essential for growth on GlcNAc ( Fig. 6a ), and transcriptional induction of GlcNAc catabolic genes ( Fig. 6b ). The defect of the rep1 mutant in GlcNAc signalling is not due to a lack of NGS1 expression ( Supplementary Fig. 6a ). Rep1 is tagged with myc at the C-terminus and is functional ( Supplementary Fig. 1b ). ChIP of Rep1-myc showed that Rep1 was present at the promoter region of NAG1 and DAC1 in a GlcNAc-independent manner, like Ngs1 ( Fig. 6c ). Immunoprecipitation of Rep1-myc showed that Rep1 could interact with Ngs1 in cells grown in either glucose or GlcNAc medium ( Fig. 6d ). Furthermore, the promoter recruitment of Ngs1 was dramatically reduced in the rep1 mutant ( Fig. 6e ), and GlcNAc-inducible H3K9 and H3K14 acetylation at the promoter chromatin was abolished in the rep1 mutant ( Supplementary Fig. 6b ). These results suggest that the Rep1 transcription factor recruits Ngs1 to the promoters of GlcNAc catabolic genes. Different from the ngs1 mutant, the rep1 mutant was also unable to grow on galactose ( Fig. 6a ). This suggests that Rep1 is not only the transcription factor for GlcNAc signalling, but also for galactose signalling. 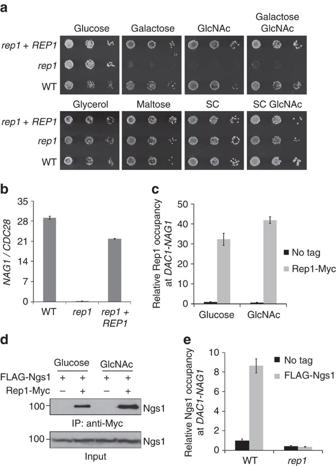Figure 6: Rep1 recruits Ngs1 to the promoters of GlcNAc catabolic genes. (a)REP1is required for growth on GlcNAc and galactose inC. albicans. Dilutions of therep1Δ/rep1Δmutant (YLO141),rep1Δ/rep1Δ::REP1(YLO142), and the wild type (SC5314) cells were spotted onto YNB solid medium containing 2.5 mM of the indicated sugar or 5% glycerol. Cells were also tested for growth on SC solid medium in the absence or presence of 2.5 mM GlcNAc. Photographs were taken after 2 days of growth at 30 °C. (b) qRT-PCR analysis ofNAG1transcription upon GlcNAc induction. Cells of the above three strains were grown in liquid SC medium with 2.5 mM GlcNAc for 2 h at 30 °C for RNA extraction. (c) ChIP of Rep1 at the promoter ofNAG1andDAC1. Therep1mutant strain expressing Rep1-Myc or untagged Rep1 was grown in SC medium with GlcNAc or glucose at 30 °C, and cells were collected at 30 min for the ChIP experiment. The ratio ofNAG1-DAC1promoter IP (bound/input) versusACT1promoter IP (bound/input) inrep1mutant cells carrying untagged Rep1 in glucose medium was set to 1.00. (d) Ngs1 interacts with Rep1. Protein lysates from strains HLY4454 (FLAG-Ngs1, Rep1-Myc) and HLY4402 (FLAG-Ngs1) were subjected to immunoprecipitation with anti-Myc antibody, and the precipitated proteins were probed with anti-FLAG antibody. As an input control, cell lysates were analysed by Western blotting with the anti-FLAG antibody. (e) Ngs1 association at theNAG1-DAC1promoter depends on Rep1. For ChIP of Ngs1 in the wild-type strain (HLY4459) or therep1mutant (HLY4453), cells were grown in SC GlcNAc medium at 30 °C for 30 min. The ratio ofNAG1-DAC1promoter IP (bound/input) versusACT1promoter IP (bound/input) in wild-type cells carrying untagged Ngs1 was set to 1.00. All data showed the average of three independent qPCR data with error bars representing the s.d. Figure 6: Rep1 recruits Ngs1 to the promoters of GlcNAc catabolic genes. ( a ) REP1 is required for growth on GlcNAc and galactose in C. albicans . Dilutions of the rep1Δ/rep1Δ mutant (YLO141), rep1Δ/rep1Δ::REP1 (YLO142), and the wild type (SC5314) cells were spotted onto YNB solid medium containing 2.5 mM of the indicated sugar or 5% glycerol. Cells were also tested for growth on SC solid medium in the absence or presence of 2.5 mM GlcNAc. Photographs were taken after 2 days of growth at 30 °C. ( b ) qRT-PCR analysis of NAG1 transcription upon GlcNAc induction. Cells of the above three strains were grown in liquid SC medium with 2.5 mM GlcNAc for 2 h at 30 °C for RNA extraction. ( c ) ChIP of Rep1 at the promoter of NAG1 and DAC1 . The rep1 mutant strain expressing Rep1-Myc or untagged Rep1 was grown in SC medium with GlcNAc or glucose at 30 °C, and cells were collected at 30 min for the ChIP experiment. The ratio of NAG1-DAC1 promoter IP (bound/input) versus ACT1 promoter IP (bound/input) in rep1 mutant cells carrying untagged Rep1 in glucose medium was set to 1.00. ( d ) Ngs1 interacts with Rep1. Protein lysates from strains HLY4454 (FLAG-Ngs1, Rep1-Myc) and HLY4402 (FLAG-Ngs1) were subjected to immunoprecipitation with anti-Myc antibody, and the precipitated proteins were probed with anti-FLAG antibody. As an input control, cell lysates were analysed by Western blotting with the anti-FLAG antibody. ( e ) Ngs1 association at the NAG1-DAC1 promoter depends on Rep1. For ChIP of Ngs1 in the wild-type strain (HLY4459) or the rep1 mutant (HLY4453), cells were grown in SC GlcNAc medium at 30 °C for 30 min. The ratio of NAG1-DAC1 promoter IP (bound/input) versus ACT1 promoter IP (bound/input) in wild-type cells carrying untagged Ngs1 was set to 1.00. All data showed the average of three independent qPCR data with error bars representing the s.d. Full size image Ngs1 also functions in other GlcNAc-induced transcription Having determined the essential role of Ngs1 in GlcNAc sensing and transcriptional activation of GlcNAc catabolic genes, we then investigated whether Ngs1 plays a role in GlcNAc-induced hyphal development. The ngs1 hxk1 double mutant was constructed and used to examine the function of Ngs1 in hyphal growth because GlcNAc is inhibitory to the growth of the ngs1 mutant at 37 °C ( Supplementary Fig. 7 ). The hxk1 mutant can grow and develop hyphae as wild type in GlcNAc containing media where GlcNAc is not the only carbon source [26] . The fact that the inhibitory effect could be removed by HXK1 deletion suggested that the reported increase in HXK1 expression at 37 °C (ref. 49 ) might lead to the accumulation of GlcNAc-6-PO 4 in the ngs1 mutant, resulting in growth inhibition as reported for the dac1 or nag1 mutants [26] ( Supplementary Fig. 7 ). Hyphal growth was induced by directly adding GlcNAc or serum into log-phase cultures to avoid inoculation-induced hyphal initiation [50] . The wild-type strain developed extensive filaments after 3.5 h of hyphal induction by serum or GlcNAc. ngs1 single mutant and ngs1 hxk1 double mutant cells also developed hyphae in serum similar to the wild-type strain ( Fig. 7a ). However, the ngs1 hxk1 double mutant displayed defective hyphal development in response to GlcNAc with a mixture of short heterogeneous filaments and over 70% yeast cells ( Fig. 7a ). Furthermore, although a slightly higher level of hyphal formation was observed in the ngs1 hxk1 double mutant upon GlcNAc induction, the expression of hypha-specific genes, such as ECE1 and HWP1 , were not induced in the double mutant ( Fig. 7b ), which may reflect the transcription-independent hyphal morphogenesis reported by Naseem et al . [17] . The ngs1 hxk1 double mutant in yeast condition displayed yeast form with a low percentage (about 20%) of germ tube, a phenotype in agreement with a previous report that deletion of HXK1 caused a high tendency to form hyphae [49] . Therefore, Ngs1 is important for GlcNAc-induced hyphal development, especially hyphal transcription. 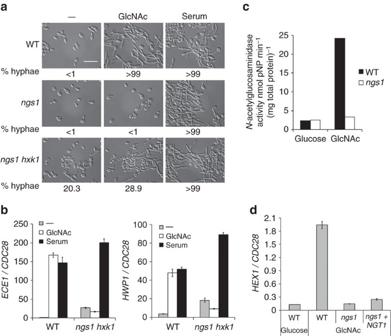Figure 7: Ngs1 is essential for GlcNAc-induced hyphal transcription andHEX1expression. Morphology (a) and qRT-PCR analysis (b) of indicated strains during hyphal induction. Cells of wild type (SC5314),ngs1(HLY4391) andngs1 hxk1double mutant (HLY4427) were grown to log phase at 30 °C, and then treated with either 50 mM GlcNAc or 10% serum. Cells were collected after incubation for 3.5 h at 37 °C. The percentage of hyphal cells was determined by counting at least 200 cells per sample. The average length of hyphae was measured to show the difference between wild type andngs1 hxk1double mutant in response to GlcNAc. Wild-type cells formed long hyphae after 3.5 h growth in GlcNAc-containing medium (46.4±12.9 μm; mean±s.d.). Hyphae length of thengs1 hxk1double mutant was shorter, 15.6±5.1 μm (mean±s.d.) in the medium without GlcNAc and 23.7±9.3 μm (mean±s.d.) upon GlcNAc induction. For all images: Scale bar, 20 μm. Expression level ofECE1andHWP1was quantified by qRT-PCR and normalized withCDC28. (c) The effect ofNGS1on GlcNAc-inducedN-acetylglucosaminidase activity inC. albicanscells. Wild type (SC5314) andngs1mutant (HLY4391) cells were resuspended in YEP medium containing 50 mM GlcNAc or glucose at OD600=0.3, andN-acetylglucosaminidase activity was measured after incubation at 30 °C for 2 h. Enzyme activities are the means of three determinations that did not vary more than 15%. (d) Expression analysis ofHEX1. Cells of wild type (SC5314),ngs1mutant (HLY4396), as well asngs1mutant carryingNGT1under theADH1promoter (HLY4393) were incubated in liquid SC medium with 2.5 mM GlcNAc or glucose for 2 h at 30 °C.HEX1expression levels were quantified by qRT-PCR and normalized withCDC28. All data showed the average of three independent qRT-PCR experiments with error bars representing the s.d. Figure 7: Ngs1 is essential for GlcNAc-induced hyphal transcription and HEX1 expression. Morphology ( a ) and qRT-PCR analysis ( b ) of indicated strains during hyphal induction. Cells of wild type (SC5314), ngs1 (HLY4391) and ngs1 hxk1 double mutant (HLY4427) were grown to log phase at 30 °C, and then treated with either 50 mM GlcNAc or 10% serum. Cells were collected after incubation for 3.5 h at 37 °C. The percentage of hyphal cells was determined by counting at least 200 cells per sample. The average length of hyphae was measured to show the difference between wild type and ngs1 hxk1 double mutant in response to GlcNAc. Wild-type cells formed long hyphae after 3.5 h growth in GlcNAc-containing medium (46.4±12.9 μm; mean±s.d.). Hyphae length of the ngs1 hxk1 double mutant was shorter, 15.6±5.1 μm (mean±s.d.) in the medium without GlcNAc and 23.7±9.3 μm (mean±s.d.) upon GlcNAc induction. For all images: Scale bar, 20 μm. Expression level of ECE1 and HWP1 was quantified by qRT-PCR and normalized with CDC28 . ( c ) The effect of NGS1 on GlcNAc-induced N -acetylglucosaminidase activity in C. albicans cells. Wild type (SC5314) and ngs1 mutant (HLY4391) cells were resuspended in YEP medium containing 50 mM GlcNAc or glucose at OD 600 =0.3, and N -acetylglucosaminidase activity was measured after incubation at 30 °C for 2 h. Enzyme activities are the means of three determinations that did not vary more than 15%. ( d ) Expression analysis of HEX1 . Cells of wild type (SC5314), ngs1 mutant (HLY4396), as well as ngs1 mutant carrying NGT1 under the ADH1 promoter (HLY4393) were incubated in liquid SC medium with 2.5 mM GlcNAc or glucose for 2 h at 30 °C. HEX1 expression levels were quantified by qRT-PCR and normalized with CDC28 . All data showed the average of three independent qRT-PCR experiments with error bars representing the s.d. Full size image Recently, it has been shown that C. albicans can obtain GlcNAc during organ colonization by secreting Hex1 as a carbon scavenger [14] . GlcNAc induces the expression of HEX1 , which encodes a secreted N -acetylglucosaminidase [51] , [52] . We detected N -acetylglucosaminidase activity in cells exposed to GlcNAc, and the activity was abolished by deletion of NGS1 ( Fig. 7c ). Since N -acetylglucosaminidase activity in C. albicans was shown to be Hex1-dependent and GlcNAc inducible [51] , we reasoned that the Ngs1-dependent and GlcNAc inducible N -acetylglucosaminidase activity we detected in C. albicans was due to Ngs1-mediated transcriptional induction of HEX1 expression. RT-PCR analysis showed that no significant induction of HEX1 was observed in the ngs1 mutant in GlcNAc medium ( Fig. 7d ). Further, overexpression of NGT1 was unable to promote HEX1 expression in the ngs1 mutant in GlcNAc. Thus, Ngs1-mediated intracellular GlcNAc signal transduction also controls HEX1 expression. GlcNAc is ubiquitously present as a component of the cell surface on a wide range of cells from bacteria to humans. To utilize the GlcNAc in the biosphere, microbes have developed various strategies for GlcNAc scavenging and utilization. Some microbes have even evolved to link GlcNAc signalling with cell fate development and virulence properties. Central to GlcNAc metabolism is how microbes sense GlcNAc in the environment and respond with a proper transcriptional program. For bacteria, extracellular GlcNAc is taken into cells using a phosphotransferase system that converts GlcNAc to GlcNAc-6-PO 4 (ref. 1 ). Intracellular GlcNAc-6-PO 4 regulates the expression of GlcNAc-induced genes by causing allosteric changes of a global transcriptional regulator in its binding affinity for the target genes [2] , [53] , [54] . Fungi use the GlcNAc transporter Ngt1 of the major facilitator superfamily transporters for GlcNAc uptake [3] , [4] , [6] . Here we show that C. albicans uses Ngs1 as the master regulator of GlcNAc signalling that can sense intracellular GlcNAc via its N-terminal GlcNAc binding domain. The GlcNAc-binding is necessary for chromatin histone acetylation through its C-terminal GNAT domain. Ngs1 controls not only the induction of GlcNAc catabolic genes; it also controls GlcNAc-induced expression of NGT1 , HEX1 and hyphal genes, which are for GlcNAc uptake, scavenging and pathogenesis, respectively ( Fig. 8 ). Targeting of Ngs1 to specific promoters is mediated through the transcriptional factor Rep1. Both Ngs1 and Rep1 are conserved in fungi, and their homologues are required for GlcNAc signalling and catabolism in the filamentous fungus T. reesei [6] . The C. tropicalis Ngs1 has the same function and regulation. Therefore, the GlcNAc signalling pathway in fungi consists of the transporter Ngt1, the sensor-transducer Ngs1, and the transcription factor Rep1/Ron1 ( Fig. 8 ). The evolution of GlcNAc regulation of promoter histone acetylation in fungi, in comparison to direct regulation of transcription factor affinity on promoter DNA in bacteria, probably reflects the need to overcome the repressive barrier imposed by the chromatin in eukaryotes. 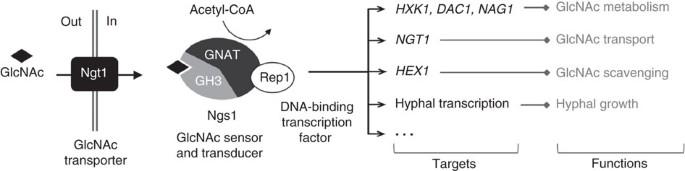Figure 8: Model of GlcNAc signalling inC. albicans. GlcNAc enters the cell via the GlcNAc-specific transporter Ngt1 (ref.3). Ngs1 acts as the sensor and signal transducer via its N-terminal GlcNAc binding domain and C-terminal GNAT domain, as well as the transcription factor Rep1 for promoter targeting. Binding of GlcNAc to Ngs1 activates theN-acetyltransferase activity, resulting in promoter histone acetylation and transcription of all GlcNAc-induced genes. Figure 8: Model of GlcNAc signalling in C. albicans. GlcNAc enters the cell via the GlcNAc-specific transporter Ngt1 (ref. 3 ). Ngs1 acts as the sensor and signal transducer via its N-terminal GlcNAc binding domain and C-terminal GNAT domain, as well as the transcription factor Rep1 for promoter targeting. Binding of GlcNAc to Ngs1 activates the N -acetyltransferase activity, resulting in promoter histone acetylation and transcription of all GlcNAc-induced genes. Full size image There is growing evidence that the molecular scaffolds employed by enzymes of sugar metabolism are ideally suited to function as ligand sensors in transcriptional regulation. For example, the Gal3 transducer of the GAL regulon in S. cerevisiae has ∼ 90% sequence similarity to galactokinase Gal1, but does not possess galactokinase activity. Gal3 interacts with the Gal80 repressor only when Gal3 is in a ‘closed’ state induced by galactose binding [55] . Another example is the negative transcriptional regulator NmrA in Aspergillus nidulans. The structure of NmrA shows unexpected similarity to a superfamily of short-chain dehydrogenase/reductases [56] . Similarly, NmrA has lost the conserved catalytic residue for enzyme activity, but appears to have adapted to use the scaffold for transcriptional regulation. The N-terminal domain of Ngs1 is very similar in structure to bacterial NagZs of the single-domain GH3 β - N -acetylglucosaminidases [34] . The binding coordinates of NagZs for GlcNAc are conserved in Ngs1 (ref. 36 ), and the interaction of Ngs1 with GlcNAc is essential for GlcNAc signalling in C. albicans . The GlcNAc binding domain is conserved in Ngs1 orthologs in fungi. Like Gal3 and NmrA, Ngs1 lacks hydrolase activity, and the conserved catalytic residues in NagZs are lost in Ngs1 and not required for GlcNAc signalling in C. albicans . We propose that Ngs1 does not function as a hydrolase in C. albicans . Rather, the conserved GlcNAc binding domain in Ngs1 functions as a GlcNAc sensor that modulates the activity of Ngs1 upon GlcNAc binding. Ngs1 is a new member of the GCN5-related N -acetyltransferase (GNAT) family. The conserved sites for Acetyl-CoA binding in the GNAT domain of Ngs1 are required for GlcNAc signalling and H3K9 and H3K14 acetylation at the promoter of GlcNAc catabolic genes. Ngs1 is a unique GNAT because its activity is induced by GlcNAc. In C. albicans , Gcn5 is responsible for almost all of acetylation at H3K9, but it is not required for GlcNAc-induced H3K9 acetylation at the promoters of GlcNAc catabolic genes. GlcNAc-induced H3K9ac is only detected at specific promoters, but not detectable when assayed with total histone, even in gcn5 mutant cells where the basal H3K9ac is low. This is likely due to a lack of a structural determinant necessary for acceptor substrate specificity in Ngs1. In support of this, the GNAT domain of Ngs1 is capable of increasing the total level of H3K9ac in response to GlcNAc when its C-terminus is replaced with the bromodomain and an Ada2 interaction domain of Gcn5. These domains of Gcn5 may allow the integration of the chimeric protein into the SAGA and ADA HAT complexes to acetylate nucleosomal histones. Recruitment of Ngs1 by Rep1 to the promoters of GlcNAc-inducible genes targets Ngs1 to specific locations for chromatin histone acetylation. Therefore, we suggest that GlcNAc-induced chromatin H3 acetylation by Ngs1 is limited to specific chromatin locations bound with Rep1. As ngs1 and rep1 mutants showed same defects, the major function of Ngs1 in GlcNAc signalling should be chromatin histone acetylation and transcriptional regulation, although we cannot exclude the possibility of Ngs1 acetylating other proteins or small molecules. Like Gcn5 (ref. 10 ) and NatA (ref. 57 ), complex formation may be necessary for Ngs1 in substrate selection. Interestingly, the domain layout in Ngs1 is similar to the mammalian O-GlcNAcase (OGA), which is responsible for removal of O-linked GlcNAc from nucleocytoplasmic proteins. Like Ngs1, OGA has a glycoside hydrolase (GH) domain at the N-terminus and a GNAT-like fold at the C-terminus [58] . However, the OGA activity resides in the GH domain and its GNAT domain has lost some conserved sites for Acetyl-CoA binding. Therefore, Ngs1 is conserved in fungi, but not in multicellular organisms. It is the first GNAT found to respond directly to the availability of a sugar in the environment and control cellular transcriptional programs. Rep1 is required for GlcNAc signalling and gene expression, as reported for Ron1 in the filamentous fungus T. reesei [6] . We demonstrate that Rep1 is the DNA-binding transcription factor that recruits Ngs1 to specific promoters for GlcNAc-induced histone acetylation and transcription. Interestingly, Rep1 is also required for galactose utilization, and GlcNAc can induce the expression of galactose metabolic genes in C. albicans [26] . The galactose signalling pathway is rewired in C. albicans and is not regulated by the Gal3, Gal80 and Gal4 regulatory circuitry [59] . In fact, the growth defect of the rep1 mutant is stronger than known mutants involved in galactose signal transduction [59] , [60] . Unlike the rep1 mutant, the ngs1 mutant can grow on galactose. This indicates that Rep1 can recruit other regulators for galactose signalling in C. albicans. Ngs1 represents the first example of how one protein can sense the availability of a sugar taken from outside the cell and directly regulate transcription by modulating its GNAT activity. The GlcNAc sensor-transducer is a master regulator of GlcNAc signalling in fungi that controls GlcNAc catabolism, morphogenesis and pathogenesis. Media and growth conditions C. albicans strains were routinely grown at 30 °C in YPD (2% Bacto peptone, 2% glucose, 1% yeast extract). Transformants were selected on synthetic medium (0.17% Difco yeast nitrogen base w/o ammonium sulphate, 0.5% ammonium sulphate and auxotrophic supplements) with 2% glucose. The ability of cells to grow was tested by spotting dilutions of cells onto YNB (0.17% Difco yeast nitrogen base w/o ammonium sulphate, 0.5% ammonium sulphate) or SC (0.17% Difco yeast nitrogen base w/o ammonium sulphate, 0.5% ammonium sulphate, complete supplement mixture of amino acids) solid media with 2.5 mM of different sugars followed by incubation at 30 °C for 2 days. To determine the expression of GlcNAc catabolic genes, cells were grown overnight in liquid YPD at 30 °C, pelleted, washed three times in PBS, diluted 1:50 in SC medium with different sugars, and incubated for 2 h at 30 °C. Hyphal development is induced in cells growing in log phase without inoculation to block the effect of farnesol depletion on hyphal induction as described previously [26] . C. albicans cells grown overnight at 30 °C in YPD were washed three times with PBS, resuspended in an equal volume of PBS, and diluted 1:100 into liquid SC medium containing 50 mM galactose. After 4 h of incubation at 30 °C, hyphal growth was induced by a shift in temperature to 37 °C in combination with 50 mM GlcNAc. In addition to GlcNAc, 10% Serum was used for morphology assay in this study as well. Screening for mutants defective in growth on GlcNAc The deletion mutant library affecting 674 genes of C. albicans [24] and the wild type reference strain SN250 were grown overnight in liquid YPD at 30 °C. Then cells were diluted 1:200 fold into sterile PBS in 96-well plates. The ability of cells to grow on different sugars was tested by spotting diluted cells onto YNB solid media with 2.5 mM glucose or 2.5 mM GlcNAc followed by incubation at 30 °C. The medium was supplemented with 0.1 mg ml −1 arginine to permit the growth of mutant strains in library. Three mutants could not grow on the GlcNAc-containing medium. However, these three mutants were able to grow to the same extent as the wild-type strain on glucose after incubation for 2 days. Plasmid and strain construction SC5314 genomic DNA was used as the template for all PCR amplifications of C. albicans genes. The C. albicans strains used in the present study are listed in Supplementary Table 2 . The primers used for PCR amplification are listed in Supplementary Table 1 . C. albicans ARG4 was amplified with primers as previously described [61] , and then transformed into the ngs1 mutant strain [24] . Transformants were selected on arginine dropout medium. Arg + transformants (HLY4391) were streaked onto 5-fluoroorotic acid plates to select for the Ura – strain (HLY4392). pBES116-NGS1 was constructed by inserting a 3.78-kb PCR fragment (primers 1 and 2) containing the NGS1 promoter and coding sequence into the NotI-PstI site of pBES116 (ref. 62 ). AscI-digested pBES116-NGS1 was introduced into ngs1 mutant (HLY4392) to express NGS1 under the endogenous promoter. Two-step PCR was used to create pBES116-NGS1 D74A . Two pairs of primers (primers 1 and 3, 2 and 4) were used to PCR amplify overlapping NGS1 fragments with the mutation in the overlapping region. The PCR products were purified and mixed as templates for another round of PCR amplification using the primers 1 and 2, which produced the full-length NGS1 D74A sequence. The resulting mutant, NGS1 D74A , was inserted into the NotI-PstI site of pBES116 to generate pBES116-NGS1 D74A . The plasmid was digested with AscI for integration into the ADE2 locus. This two-step PCR procedure was used to introduce mutations into NGS1 in a pBES116-based construct. Mutations were confirmed by sequencing. Plasmids for expression of 3 × FLAG tag fusion proteins were constructed as follows. The promoter region of NGS1 was amplified with primers 1 and 23 and inserted into the NotI-PstI site of pBES116 to generate pBES116-NGS1p. PCR products (primers 24 and 2) containing the entire NGS1 coding region and a 3 × FLAG tag were amplified from constructs pBES116-NGS1 and pBES116-NGS1 with mutations. The DNA fragments were then inserted into pBES116-NGS1p at the PstI site. The resulting plasmids were digested with AscI and introduced into ngs1 mutant strain (HLY4392) to express the 3 × FLAG fusion proteins under the endogenous promoter. A 2.9-kb PCR product (primers 27 and 28) containing the entire NGS1 coding region was inserted into the MluI site of Mal2-GFP-HGC1 (ref. 61 ) to create MAL2p-GFP-NGS1. The AscI-digested MAL2p-GFP-NGS1 DNA fragment was introduced into the ngs1 mutant strain (HLY4392) for GFP-Ngs1 expression. A 1.91-kb PCR product (primers 1 and 31) containing the NGS1 promoter and N-terminal NGS1 coding region was inserted into the NotI-PstI site of pBES116 to generate pBES116-NGS1N. The 3 × FLAG tagged N-terminal NGS1 was amplified with primers 24 and 31 and inserted into pBES116-NGS1p at the PstI site. The C-terminal NGS1 coding region was amplified using primers 32 and 33. The resulting PCR product was digested with PstI and KpnI and inserted into the PstI-KpnI site of pBES116-NGS1p to create pBES116-NGS1C. To express 3 × FLAG fusion protein, the C-terminal NGS1 was amplified using primers 44 and 33 and then ligated with pBES116-NGS1p. The NGS1 ortholog in Candida tropicalis (CTRG_01063) was obtained by PCR (primers 38 ad 39) using genomic DNA from ATCC 750. The resulting PCR product was digested with PstI and EcoRV and inserted into the pBES116-NGS1p to create pBES116-CtNGS1. Two-step PCR was used to produce pBES116-CtNGS1 KH175/176AA and pBES116-CtNGS1 G700L . To create a chimera comprising the Ngs1 GNAT domain fused to the ADA2 interaction domain and bromodomain in Gcn5, we used a strategy employing PCR-mediated recombination so that no restriction sites at the junction of the chimera are needed. Primers 46 and 47 were designed in a way that both PCR products shared the same sequence at one end. The PCR product (primers 45 and 48) corresponding to Ngs1 aa 595 to 752 plus Gcn5 aa 253 to 450 was inserted into the BamHI-MluI site of pPR671-SAT1 (ref. 63 ) to create pPR671-chimera-SAT1. The SacI-digested pPR671-chimera-SAT1 fragment was integrated into the NGS1 locus in the gcn5 mutant. The REP1 coding sequence (primers 49 and 50) was inserted into the BamHI-MluI site of pPR671-SAT1 and p673 (ref. 64 ) to generate plasmids pPR671-REP1-SAT1 and pPR673-REP1. The resulting constructs were digested with StuI to integrate into the genomic RP10 locus for expression of 13 × Myc fusion proteins under the ACT1 promoter. NGT1 was deleted using SAT1 -flipping strategy [65] . Upstream (primers 13 and 14) and downstream (primers 15 and 16) sequences of NGT1 were cloned as ApaI-XhoI and NotI-SacII fragments, respectively, on both sides of the SAT1 flipper cassette to obtain the plasmid pSFS2-NGT1 for NGT1 disruption. To disrupt the endogenous copies of NGT1 in wild-type cells, pSFS2-NGT1 was linearized using ApaI and SacII, which was followed by two sequential rounds of transformation, selection, and recycling of the SAT1 marker. pBA1-NGT1 was constructed for expression of NGT1 under the control of ADH1p in C. albicans . The full-length coding sequence of NGT1 was amplified with primers 25 and 26 and inserted into the ClaI-KpnI site of pBA1 (ref. 66 ) to generate pBA1-NGT1. HXK1 deletion in ngs1 mutant strain was based on PCR recombination by the method of Wilson et al . [67] . Primers 34 and 35 were used to amplify C . albicans URA3 and ARG4 from plasmids pGEM-URA3 and pRS-ARG4ΔSpeI, respectively. The ngs1 mutant strain [24] was streaked onto 5-fluoroorotic acid plates to select for the Ura – strain. The first copy of HXK1 was disrupted by the transformation of ARG4 into the ngs1 mutant (Ura – ) strain. C. albicans URA3 was used to replace the second copy of HXK1 . All deletions were confirmed by PCR. Microscopy Cells of ngs1 mutant carrying GFP-Ngs1 under the MAL2 promoter and wild-type strain were grown overnight to log phase in liquid SC medium containing 50 mM maltose, and then treated with or without 50 mM GlcNAc for 30 min. GFP-Ngs1 was detected by fluorescence microscopy, and cell morphology was detected using differential interference contrast (DIC) optics. Images were obtained on an inverted Zeiss Axio Observer.Z1 microscope (Carl Zeiss MicroImaging, Inc., Thornwood, NY) fluorescent system equipped with an X-Cite series 120 mercury lamps. DAPI (4′,6-diamidino-2-phenylindole) stain was applied for the visualization of the cell nucleus. Each photomicrograph represents the majority of the cells. Quantitative PCR expression analysis Total RNA was purified from C. albicans cells using the RNeasy Mini kit and DNase-treated at room temperature for 15 min using the RNase-free DNase Set (Qiagen), cDNA was synthesized using the SuperScript II Reverse Transcriptase kit (Invitrogen), and qPCR was done using the iQ SYBR Green Supermix (Bio-Rad). The primers for HXK1 , DAC1, NGT1 and NAG1 were used as previously described [26] . Primers for HWP1 and ECE1 were used as described by Lu et al . [64] . Primers for HEX1 were used as described by Ruhela et al . [14] . Primers 51 and 52 were used to amplify C . albicans NGS1. Primers 29 and 30 were used to amplify C . albicans CDC28. The signals obtained from CDC28 mRNA were used for normalization. All data showed the average of three independent qRT-PCR experiments with error bars representing the s.d. Chromatin immunoprecipitation Cells were grown overnight in liquid YPD at 30 °C, pelleted, washed three times in PBS, diluted 1:20 in SC medium supplemented with 10 mM GlcNAc or glucose, and collected at 30 min for Chromatin immunoprecipitation. ChIP experiments were performed as described with modifications [63] . DNA was sheared by sonication eight times for 20 s at high power on a Bioruptor (diagenode) with 40 s intervals. For the IP, 5 μl of anti-FLAG (F3165, Sigma), 10 μl of anti-Myc (SC-789, Santa Cruz), 4 μl of anti-H3 (ab1791, Abcam), 5 μl of anti-acetylated-H3K9 (06-942; Millipore) or 5 μl of anti-acetylated-H3K14 (ab52946; Abcam) antibodies were used for ∼ 2 mg of chromatin proteins in an immunoprecipitation volume of 300 μl. ChIP DNA was quantitated by qPCR with primers 17 and 18 at the promoter for DAC1 and NAG1 . The ACT1 promoter (primers 36 and 37) served as a negative control. FLAG-Ngs1 and Rep1-Myc expressing strains were used with untagged strains as controls. The FLAG-Ngs1 or Rep1-Myc enrichment is presented as a ratio of NAG1-DAC1 promoter IP (bound/input) versus control locus IP (bound/input). H3 ChIP signal was used to normalize H3K9ac and H3K14ac values. Levels of H3K9ac and H3K14ac at the NAG1-DAC1 promoter were further normalized to the respective value at the ACT1 promoter region. The ChIP data showed the average of three independent qPCR data with error bars representing the s.d. N -acetylglucosaminidase assay N -acetylglucosaminidase activity was measured in whole cell extracts, using pNP-β-D-GlcNAc (4-Nitrophenyl N-acetyl-β-D-glucosaminide, Sigma) as a substrate. Overnight cultures of wild-type and ngs1 mutant cells were washed three times in sterile PBS, resuspended in YEP (2% Bacto peptone, 1% yeast extract) medium containing 50 mM GlcNAc or glucose at OD 600 =0.3, and incubated at 30 °C for 2 h. Cells of each sample were pelleted at 3,000 g for 5 min at 4 °C, and resuspended in 0.35 ml of lysis buffer (50 mM Tris–HCl, pH 7.5, 150 mM NaCl, 0.1% NP40) plus protease inhibitor cocktail (Roche). Total protein was extracted using a Fast-Prep system (FastPrep-24; MP Biomedicals). Protein concentration was determined by the Bradford method. Equal amounts of proteins were incubated at 37 °C for 30 min in 0.25 ml volumes containing the following: 1 mg ml −1 pNP-β-D-GlcNAc, 50 mM sodium phosphate buffer, pH 5.5 and 50 mM NaCl. Reactions were stopped by the addition of 0.5 ml of 4% (wt per vol) Na 2 CO 3 , and the absorbance was measured at 405 nm. An extinction coefficient of 18,300 (M × cm) −1 was used to calculate p -nitrophenol produced per minute. One unit of enzyme was defined as that which catalysed the formation of 1 μmol of p -nitrophenol per min. No hydrolysis of pNP-β-D-GlcNAc was detected in the controls, containing boiled extracts of C. albicans cells. GlcNAc-agarose affinity chromatography A total of 400 μl of protein extract from cells expressing wild-type or mutant 3FLAG-Ngs1 or untagged Ngs1 was incubated with 50 μl GlcNAc-agarose beads (A2278; Sigma) overnight at 4 °C under rotation. The beads were washed three times with TBS buffer (20 mM Tris-HCl, pH 7.5, 150 mM NaCl) to remove unbound protein. The bound protein was eluted from the matrix with 50 μl of 4% SDS for 30 min at 23 °C. The samples were collected by low-speed centrifugation. The input and bound fractions were analysed on Western blots. Uncropped scans of western blots are presented in Supplementary Fig. 8 . Data availability The authors declare that all data supporting the findings of this study are available within the article and its Supplementary Information , or from the corresponding author on request. How to cite this article: Su, C. et al . N-acetylglucosamine sensing by a GCN5-related N -acetyltransferase induces transcription via chromatin histone acetylation in fungi. Nat. Commun. 7, 12916 doi: 10.1038/ncomms12916 (2016).